Bottom-up synthesis of finite models of helical (n,m)-single-wall carbon nanotubes The bottom-up synthesis of hoop-shaped aromatic hydrocarbons is currently attracting interest, because they can serve as finite models of single-wall carbon nanotubes (SWNTs). Models for chiral ( n,m )-SWNTs, particularly those with optical activity, have not been synthesized but are of special interest owing to their anomalous helical network of sp 2 -carbons. Here we show that finite model compounds for (12,8)-, (11,9)- and (10,10)-SWNTs are synthetically accessible by a stepwise macrocyclization of [4]phenacene, a compound that bears fused benzene rings in a zigzag arrangement, and we can isolate and identify all the isomers including the enantiomers with ( P )- and ( M )-helicity. The complete isolation and identification of the model compounds led to the first examination of the stereo-disproportionation of chiral SWNT models, which encourages the future studies on asymmetric induction for the synthesis. Bottom-up synthesis of hoop-shaped aromatic hydrocarbons is currently attracting great interest because of both the difficulty with which these compounds are synthesized and the fact that they contain tubular structures that can serve as finite models of single-wall carbon nanotubes (SWNTs). Although the synthesis of finite models for armchair ( n,n )-SWNTs has been intensely investigated with cycloparaphenylenes (CPP) over the past few years [1] , [2] , [3] , [4] , [5] , [6] , the synthesis and isolation of models for chiral ( n,m )-SWNTs ( n ≠ m ), particularly those bearing persistent structures with optical activity, has not been achieved. The chiral ( n,m )-SWNT models are intriguing targets, possessing chirality inherent to the anomalous helical arrangements of the sp 2 -carbon network; however, many issues arise in the synthesis, isolation and characterization of such compounds. A recent investigation of the synthesis of a (15,14)-SWNT model further exemplifies another serious issue: a loss of optical activity with CPP congeners may arise because of racemization by rotation around the single-bond linkages under ambient conditions [7] . Here we report the synthesis of [4]cyclo-2,8-chrysenylene ([4]CC), a macrocyclic tetramer of chrysene ([4]phenacene) molecules that are linked by four single bonds. We found that we could isolate a complete set of rotational isomers of the cyclophenacenylenes, including the helical enantiomers, and fully characterize the persistent rigid tubular structures that serve as finite models for ( P )/( M )-(12,8)-SWNTs, ( P )/( M )-(11,9)-SWNTs and (10,10)-SWNTs [8] . Notably, the present synthesis is the first example of the bottom-up construction of cyclophenacene congeners, which have previously been prepared only through top-down chemical synthesis from [60]fullerene [9] . Finally, we explored the possibility of enantioenrichment in the synthesis, which may call for the further challenge of bottom-up asymmetric synthesis of single chiral SWNTs in the future. Synthesis We synthesized [4]CC through the application of biaryl homocoupling to diborylchrysene [10] . After a few unsuccessful trials of one-pot homocoupling reactions of 2,8-dibromochrysene 1 (refs 11 , 12 ), we arrived at a two-step synthesis involving the isolation of a Pt-complex as the synthetic intermediate, a strategy similar to that of the pioneering studies of Yamago for the synthesis of [8]CPP [3] , [5] . In our synthesis, we found that the arylated Pt-complex could be obtained straightforwardly through the reaction of boronate ester with divalent platinum. After converting dibromide 1 to diborylchrysene 2 , 2 was subjected to the metalation reaction with PtCl 2 (cod) in the presence of CsF to afford Pt-complex 3 in 74% yield ( Fig. 1 ; Supplementary Methods ). The structural analysis of 3 by nuclear magnetic resonance (NMR) spectroscopy indicated that chrysenylene units are freely rotating around the single-bond linkages at ambient temperature, and the square structure was established through the X-ray analysis of a single crystal ( Supplementary Fig. S1 ). The final cyclization step was then effected through a ligand exchange reaction with PPh 3 and a subsequent reductive elimination reaction at 100 °C to give [4]CC in 94% yield as a mixture of isomers [13] . 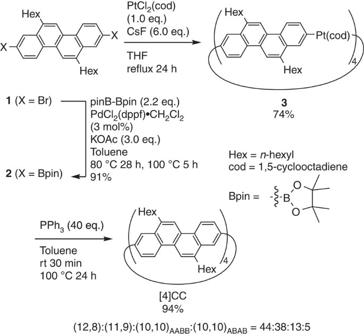Figure 1: Synthesis of [4]CC. The ratios of isomers are the molar ratios determined by HPLC analysis. Figure 1: Synthesis of [4]CC. The ratios of isomers are the molar ratios determined by HPLC analysis. Full size image Structures Before providing further experimental details, we describe the structures of the possible isomers of [4]CC to clarify the complex and challenging issues involved in its isolation and identification. Depending on the relative orientations of the chrysenylene units in the nanohoop, the total number of possible isomers of [4]CC is six, including two sets of helical enantiomers. 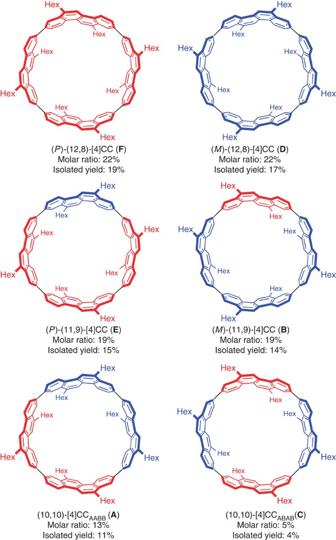Figure 2: Structures of the [4]CC isomers. The two possible chrysenylene orientations are shown in red and blue. The molar ratio was determined by HPLC analysis of a mixture of [4]CC isomers, and the yields were recorded after isolation of each isomer with preparative HPLC. All the possible structures, each of which bears a model structure for a different SWNT, are shown in Figure 2 . Using the conventional assignments of the chiral index of SWNTs [8] , we can group the isomers first into three structures: (12,8)-[4]CC, (11,9)-[4]CC and (10,10)-[4]CC. The chiral ( n,m )-isomers can be grouped further into helical enantiomers of ( P ) and ( M ), and the two different isomers of (10,10)-[4]CC can be assigned, respectively, as (10,10)-[4]CC AABB and (10,10)-[4]CC ABAB , depending on the relative orientations of chrysenylene units. Figure 2: Structures of the [4]CC isomers. The two possible chrysenylene orientations are shown in red and blue. The molar ratio was determined by HPLC analysis of a mixture of [4]CC isomers, and the yields were recorded after isolation of each isomer with preparative HPLC. Full size image Isolation We succeeded in the isolation of the complete set of six isomers using a readily available column of surface-modified silica gel. Thus, a mixture of [4]CC was subjected to reserve-phase high-pressure liquid chromatography (HPLC) using cholesterylated silica gel (COSMOSIL Cholester column) to delineate each isomer, A – F , as a separated peak ( Fig. 3a ). Although the peaks of three isomers ( A – C ) overlapped by ultraviolet-vis detection, detection with a circular dichroism (CD) method enabled us to determine the molar ratio of the six isomers ( A : B : C : D : E : F =13:19:5:22:19:22) and also to assign the isomers with helical chirality ( B , D , E , F ). Note that the separation and the CD activity unequivocally show that, unlike the previous examples of CPP [7] , the single-bond linkages in the nanohoop are rotationally constrained at ambient temperature and that all the isomers, including the helical enantiomers, were separated on the chiral steroidal stationary phase. It is interesting to note that the rotation of chrysenylene units at the single-bond linkages are restricted in the absence of any apparent steric repulsions that are requisite structural factors for the conventional restricted rotation. Exerting the chromatographic separation on a preparative scale with larger columns ( Supplementary Fig. S2 ), we obtained all the isomers in a pure form with the yields shown in Figure 2 . 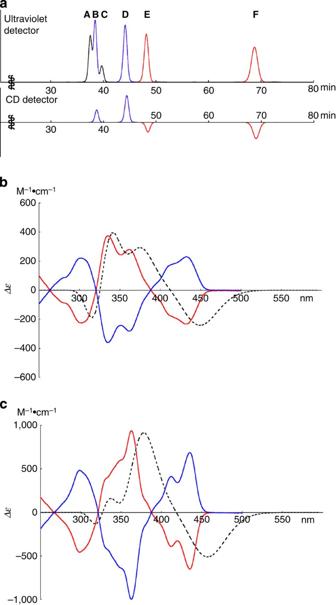Figure 3: Analysis of [4]CC isomers. (a) HPLC analysis of [4]CC using COSMOSIL Cholester columns. The top chart shows the analysis with ultraviolet-vis detection at 300 nm, and the bottom chart shows the simultaneous analysis with CD detection at 420 nm. Peaks with positive CD are shown in blue, and those with negative CD are in red. (b) Experimental and theoretical CD spectra of (12,8)-[4]CC. The plain curves in blue and red are the experimental spectra of isomersBandE, respectively. The broken curve is a theoretical spectrum of (P)-(12,8)-[4]CC with methyl substituents. (c) Experimental and theoretical CD spectra of (11,9)-[4]CC. The plain curves in blue and red are the experimental spectra of isomersDandF, respectively. The broken curve is a theoretical spectrum of (P)-(11,9)-[4]CC with methyl substituents. Figure 3: Analysis of [4]CC isomers. ( a ) HPLC analysis of [4]CC using COSMOSIL Cholester columns. The top chart shows the analysis with ultraviolet-vis detection at 300 nm, and the bottom chart shows the simultaneous analysis with CD detection at 420 nm. Peaks with positive CD are shown in blue, and those with negative CD are in red. ( b ) Experimental and theoretical CD spectra of (12,8)-[4]CC. The plain curves in blue and red are the experimental spectra of isomers B and E , respectively. The broken curve is a theoretical spectrum of ( P )-(12,8)-[4]CC with methyl substituents. ( c ) Experimental and theoretical CD spectra of (11,9)-[4]CC. The plain curves in blue and red are the experimental spectra of isomers D and F , respectively. The broken curve is a theoretical spectrum of ( P )-(11,9)-[4]CC with methyl substituents. Full size image Identification The next challenge of structural identification of the isolated isomers was accomplished by NMR spectroscopy and CD spectroscopy. As is often the case with fullerene derivatives [14] , [15] , we can assign the chiral index of [4]CC from 13 C NMR spectra by using the difference in the point symmetry of each structure. The numbers of aromatic carbon resonances, observed experimentally with the isolated isomers, were A =17, B / E =30, C =9 and D / F =9, where the two sets of CD-active isomers, B / E and D / F , displayed identical NMR spectra ( Supplementary Figs S3 and S4 ), which reveals that they are the enantiomers of the ( n,m )-isomers, respectively. Taking into account the symmetric operations inherent to each structure shown in Figure 2 , we can expect the numbers of inequivalent aromatic carbons to be the following: ( P )/( M )-(12,8)-[4]CC ( D 4 symmetry)=9, ( P )/( M )-(11,9)-[4]CC ( C 2 symmetry)=36, (10,10)-[4]CC AABB ( C 2 h symmetry)=18 and (10,10)-[4]CC ABAB ( D 4 d symmetry)=9. Combining these facts including inevitable overlaps of the observed carbon resonances, we unequivocally assigned the chiral index of the isomers as follows: (12,8)-[4]CC= D / F , (11,9)-[4]CC= B / E , (10,10)-[4]CC AABB = A and (10,10)-[4]CC ABAB = C ( Fig. 2 ). The helical handedness of ( P ) and ( M ) for the ( n,m )-isomers was further identified by CD spectroscopy and theoretical calculations [8] , [16] . As shown in Figure 3b,c , the CD spectrum of B was the mirror image of E , and the CD spectrum of D was the mirror image of F . This observation confirmed the enantiomeric relationship between these two sets of isomers. By performing time-dependent density functional theory calculations using the B3LYP/6-31G(d,p) functional, we obtained theoretical spectra for the ( P )-isomers bearing methyl substituents [17] . Matching the experimental and theoretical spectra, as shown in Figure 3b,c , we can assign isomer E as ( P )-(11,9)-[4]CC and isomer F as ( P )-(12,8)-[4]CC, which, consequently, led the assignment of isomer B as ( M )-(11,9)-[4]CC and isomer D as ( M )-(12,8)-[4]CC. With the theoretical analysis, the negative CD bands at the longest wavelengths (432 nm for E and 434 nm for F ) can be ascribed to the transition between the HOMO and the LUMO that are fully delocalized over the tubular structures ( Supplementary Fig. S7 ). Thus, the negative rotational bands from the first transition may be regarded as characteristic signatures of ( P )-helical (12,8)- and (11,9)-SWNTs. With these identifications in hand, we completed the assignments of the chiral indices for all the isomers of [4]CC, as shown in Figure 2 . It is interesting to note that both of the ( P )-isomers are retained longer in the steroidal environment of the HPLC column. Enantioenrichment The complete isolation and assignment prompted us to examine the asymmetric induction to explore the possibility of stereoselective synthesis of chiral SWNT models. However, we could not find any appropriate chiral phosphine ligands for the stereo-discrimination and realized that chrysenylene units in [4]CC can rotate at an elevated temperature, although the rotation has not been observed at ambient temperature at least for several tens of hours. Thus, when ( P )-(12,8)-[4]CC was heated at 100 °C in toluene, we started observing the other five isomers after 1 h and, after 8 h, the ratio of all the isomers reached at the same value before the separation. Although the precise energetics of the rotational barrier should be investigated in due course, we then examined the enantioenrichment in the synthesis by combining the disproportionating equilibration process with the preceding reductive elimination step. 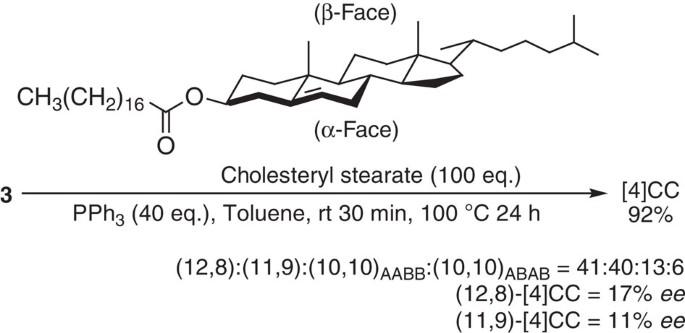Figure 4: Enantioenrichment during the synthesis of [4]CC. Enantiomers with (P)-helicity were enriched by the presence of cholesteryl stearate. The enantiomeric excesses and the ratios of isomers were determined by HPLC analysis. As shown in Figure 4 , when we carried out the reductive elimination in the presence of an excess amount of cholesteryl stearate, we obtained the ( P )-isomers of (12,8)- and (11,9)-[4]CC preferably over the ( M )-isomers and recorded enantiomeric excesses of 17% for (12,8)-[4]CC and 11% for (11,9)-[4]CC. The results show that, in the presence of the steroidal additives, [4]CC undergoes disproportionation of enantiomers at an elevated temperature, which may involve favourable interactions of steroids' α-face with the convex outer surface of the molecules [18] , [19] . The hypothesis is also supported by the fact that the isomers such as ( P )-isomers that display a steroid-like face of chrysenylene units outward (shown in red in Fig. 2 ) are preferably obtained and that these isomers also tend to remain longer in the steroidal environment of the cholesterylated silica gel. Figure 4: Enantioenrichment during the synthesis of [4]CC. Enantiomers with ( P )-helicity were enriched by the presence of cholesteryl stearate. The enantiomeric excesses and the ratios of isomers were determined by HPLC analysis. Full size image We have demonstrated that cyclophenacenylenes with single-bond linkages can maintain the hoop-shaped structure at ambient temperature and can be isolated as finite models for chiral ( n,m )-SWNTs with persistent helical chirality. Spectroscopic characteristics of the finite models should provide indispensable information for the parent SWNTs, especially in the identification of their helicity with CD spectra. This first example of enantioenrichment on the synthesis of chiral SWNT models encourages further studies in the stereoselective synthesis as well as in the use of steroids both for separations and asymmetric induction. The application of the shortest finite models as base templates for the selective synthesis of SWNTs through elongation processes is another intriguing possibility to be explored [20] , [21] , [22] , and the chemistry of [4]CC at the periphery is currently under investigation. Synthesis and characterization The synthesis of intermediate 1 was based on the protocols established for the synthesis of chrysene derivatives [10] and is reported in Supplementary Methods along with the physical data for the characterization of new compounds. Synthesis of 2 A mixture of dibromochrysene 1 (3.06 g, 5.50 mmol), bis(pinacolato)dibrone (3.07 g, 12.1 mmol), PdCl 2 (dppf)•CH 2 Cl 2 (135 mg, 165 μmol) and KOAc (1.62 g, 16.5 mmol) in toluene (32.4 ml) was stirred at 80°C for 28 h and at 100°C for 5 h. To the mixture was added water ( ca. 100 ml), and the organic materials were extracted with chloroform (4×50 ml). The organic layer was washed with brine, dried over magnesium sulfate, and concentrated in vacuo . The crude material was purified by silica gel column chromatography (eluent: 60% CHCl 3 /hexane) to afford 2 in 91% yield (3.24 g, 5.00 mmol) as a pale brown solid. Synthesis of 3 A mixture of boronate ester 2 (100 mg, 154 μmol), PtCl 2 (cod) (57.6 mg, 154 μmol) and CsF (140 mg, 924 μmol) in tetrahydrofuran (7.7 ml) was heated at reflux for 24 h. To the mixture was added water ( ca. 5 ml), and the organic materials were extracted with chloroform (4×20 ml). The organic layer was washed with brine, dried over magnesium sulfate, and concentrated in vacuo . The crude material was washed with tetrahydrofuran (ca. 30 ml) to afford 3 in 74% yield (78.8 mg, 113 μmol) as an analytically pure material Synthesis of [4]CC A mixture of platinum complex 3 (72.5 mg, 26.0 μmol) and triphenylphosphine (273 mg, 1.04 mmol) in toluene (8.67 ml) was stirred at ambient temperature for 30 min and at 100°C for 24 h. After removal of volatile materials in vacuo , the residual materials were purified by silica gel column chromatography (eluent: 20% CHCl 3 /hexane) to afford [4]CC as a mixture in 94% yield (38.5 mg, 24.4 μmol). Analysis of [4]CC isomers by HPLC A mixture of [4]CC isomers were analysed by an analytical HPLC system equipped with cholesterylated columns (COSMOSIL Cholester 4.6φ×250+250+250 mm, Nacalai Tesque; 40°C in a column oven JASCO CO-2060PLUS) under the detection with ultraviolet-vis (JASCO MD2018PLUS; 300 nm) and CD (JASCO CD-2095; 420 nm) detectors at flow rate of 1.0 ml min −1 with eluent of 60% CH 2 Cl 2 /MeOH. To deconvolute the first three peaks of A – C in the ultraviolet-vis chart, we used CD peaks of B as a reference and subtracted the adjusted peak from the ultraviolet-vis chart to obtain the corrected area ratio of all six peaks. We then converted the area ratio to the molar ratio by applying molar absorption coefficients of each isomers at the detection wavelength: (10,10)-[4]CC AABB ( A )=1.11×10 5 M −1 cm −1 , (11,9)-[4]CC ( B , E )=1.07 × 10 5 M −1 cm −1 , (10,10)-[4]CC ABAB ( C )=1.16×10 5 M −1 cm −1 , (12,8)-[4]CC ( D , F )=1.18×10 5 M −1 cm −1 . See Supplementary Fig. S5 for the ultraviolet-vis spectra. The corrected molar ratio was ( P )-(12,8)-[4]CC ( F ): ( M )-(12,8)-[4]CC ( D ) : ( P )-(11,9)-[4]CC ( E ) : ( M )-(11,9)-[4]CC ( D ) : (10,10)-[4]CC AABB ( A ) : (10,10)-[4]CC ABAB ( C )=22:22:19:19:13:5. We repeated the reaction and analysis five times and confirmed that the errors in the molar ratio are within the standard deviation of 0.5% at a maximum. Isolation of [4]CC isomers by HPLC A mixture of [4]CC isomers (38.5 mg) was separated by a recyclable HPLC system (JAI LC-908) equipped with cholesterylated columns (COSMOSIL Cholester 20φ×250+250 mm, Nacalai Tesque) under detection with a ultraviolet-vis detector at flow rate of 9.0 ml min −1 with eluent of 60% CH 2 Cl 2 /MeOH. See Supplementary Figure S2 for the HPLC charts. The mixture was first separated into three fractions (#1–#3; Supplementary Fig. S2a ), and ( P )-(12,8)-[4]CC ( F ) was obtained from the fraction #3 (7.6 mg, 19% yield). The fraction #2 was subjected to another HPLC separation ( Supplementary Fig. S2b ), and ( M )-(12,8)-[4]CC ( D ) and ( P )-(11,9)-[4]CC ( E ) were obtained after two cycles in 17% (7.1 mg) and 15% yield (6.2 mg), respectively. The fraction #1 was also subjected to another HPLC separation ( Supplementary Fig. S2c ) to afford (10,10)-[4]CC AABB ( A ), ( M )-(11,9)-[4]CC ( B ) and (10,10)-[4]CC ABAB ( C ) in 11% (4.5 mg), 14% (5.8 mg) and 4% (1.8 mg), respectively. Theoretical calculations The Gaussian 09 program suite was used in all calculations [23] , and the results, including simulated CD curves with Gaussian approximations [24] , were visualized on GaussView 5.0.9. All the calculations were performed using methyl-substituted congeners as the model and at the density functional theory (DFT) level with the B3LYP functional, the gradient correction of the exchange functional by Becke [25] , [26] and the correlation functional by Lee, Yang and Parr [27] . The 6-31G(d,p) split valence plus polarization basis set was used [28] , [29] , [30] , [31] , [32] . Cartesian coordinates for the optimized geometries are shown in Supplementary Tables S1 and S2 . Spectra calculations were performed by time-dependent DFT for the first 30 singlet–singlet transitions with an extra keyword of IOP(9/40=2) to output information on smaller contributions to each electronic transition. Note that, although the spectral analysis with the B3LYP functional yields an excellent consistence in the ordering of states with the experimental results, it tends to underestimate the excitation energy to afford slightly red-shifted theoretical spectra [17] . The spectra with convoluted curves were obtained with peak half-width of 0.15 eV at the half-height and shown in Supplementary Figure S6 . The CD signal at the longest wavelength was ascribed mainly to the HOMO–LUMO transition, and the corresponding orbitals are shown in Supplementary Fig. S7 . Enantioenrichment in the synthesis of [4]CC A mixture of platinum complex 3 (10.0 mg, 3.58 μmol), triphenylphosphine (37.5 mg, 14.3 μmol) and cholesteryl stearate (234 mg, 358 μmol) in toluene (190 μl) was stirred at ambient temperature for 30 min and at 100°C for 24 h. After removal of volatile materials in vacuo , the residual materials were purified by silica gel column chromatography (eluent: 20% CHCl 3 /hexane) to afford [4]CC as a mixture in 92% yield (5.2 mg, 3.3 μmol). The mixture was analysed by HPLC ( Supplementary Fig. S8 ), and the molar ratio of six isomers was determined as ( P )-(12,8)-[4]CC ( F ) : ( M )-(12,8)-[4]CC ( D ) : ( P )-(11,9)-[4]CC ( E ) : ( M )-(11,9)-[4]CC ( B ) : (10,10)-[4]CC AABB ( A ) : (10,10)-[4]CC ABAB ( C )=24:17:22:18:13:6. Thus, the enantiomeric excesses were 17% and 11% for ( P )-(12,8)-[4]CC and ( P )-(11,9)-[4]CC, respectively. How to cite this article: Hitosugi, S. et al . Bottom-up synthesis of finite models of helical ( n,m )-single-wall carbon nanotubes. Nat. Commun. 2:492 doi: 10.1038/ncomms1505 (2011).